Two-colour hard X-ray free-electron laser with wide tunability Ultrabrilliant, femtosecond X-ray pulses from X-ray free-electron lasers (XFELs) have promoted the investigation of exotic interactions between intense X-rays and matters, and the observation of minute targets with high spatio-temporal resolution. Although a single X-ray beam has been utilized for these experiments, the use of multiple beams with flexible and optimum beam parameters should drastically enhance the capability and potentiality of XFELs. Here we show a new light source of a two-colour double-pulse (TCDP) XFEL in hard X-rays using variable-gap undulators, which realizes a large and flexible wavelength separation of more than 30% with an ultraprecisely controlled time interval in the attosecond regime. Together with sub-10-fs pulse duration and multi-gigawatt peak powers, the TCDP scheme enables us to elucidate X-ray-induced ultrafast transitions of electronic states and structures, which will significantly contribute to the advancement of ultrafast chemistry, plasma and astronomical physics, and quantum X-ray optics. In the past few years, X-ray free-electron lasers (XFELs) [1] , [2] have stimulated to discover interesting phenomena originating from nonlinear interactions between intense X-rays and matters. These processes are mostly driven by ultrafast transition of inner-shell electrons with large energy transfers [3] , [4] , [5] . For example, Vinko et al. [4] reported creation of solid-density plasma with a temperature above 10 6 K, which has been pumped by 1.8 keV XFEL light and probed by Kα emission spectra spreading over 200 eV at photon energies around 1.6 keV. Rohringer et al. [5] found an amplification of 849 eV Kα emission from neon atoms in population inverted conditions, which are generated with irradiation of intense 960 eV XFEL light. Although these experiments have been performed by using a single XFEL beam, a two-colour double-pulse (TCDP) XFEL with a wide photon energy range and precisely controlled delay is desirable for investigating phenomena in a time–energy domain. By using the TCDP scheme, time-resolved X-ray spectroscopy of X-ray-induced phenomena will reveal mechanism and dynamics of ultrafast transition of electronic states. To obtain the information over a large spectral range, wide tunability of the X-ray probe pulse becomes essentially important. For the X-ray diffraction measurements of nanocrystals [6] , [7] and single particles [8] , the TCDP allows to investigate ultrafast structural changes, in which a large spectral separation between two pulses is indispensable for discriminating diffracted or scattered X-rays of the probe pulse from those of the pump pulse. The TCDP can also offer a method like multi-wavelength anomalous diffraction [9] . The FEL generates highly intense coherent radiation when a relativistic electron beam passes through a transverse periodic magnetic field of an undulator [10] . Since no optical cavity is practically available for X-rays, XFELs amplify and saturate radiation fields in a single pass through a long undulator, which is called a self-amplified spontaneous emission scheme (SASE) [11] , [12] . Since the FEL uses free electrons, its wavelength can be freely tuned by changing the resonant condition of the interaction between radiation fields and electrons inside the undulator. The radiation wavelength of the FEL, λ , is expressed as where λ u is the undulator periodic length, K is the undulator deflection parameter and γ is the Lorenz factor of the electron beam energy. Since the two-colour pulses are emitted from the same electron bunch, the radiation wavelength should be tuned by changing K through the strength of the undulator magnetic field. Hence variable-gap undulators are indispensable to achieve a wide spectral range in the TCDP operation. The first attempt to generate two-colour pulses in the FEL dates back to 1990s using an infrared FEL with an optical cavity [13] . Recently, two-colour FEL operations are extended to vacuum ultraviolet and soft X-ray regions [14] , [15] ; however, separation of the two wavelengths has been limited within a few per cent. In this article, we report the first TCDP operation in hard X-rays using the SPring-8 Angstrom Compact free electron LAser (SACLA) [2] , which currently covers the photon energy range between 5–15 keV by SASE. Variable-gap undulators of SACLA (see methods) enable to achieve a wide tunable range and relative wavelength separation of more than 30% in the TCDP operation. Experimental setup Since sub-10-fs pulses are routinely available in SACLA [16] , the TCDP operation with a simple and lucid scheme can achieve high temporal resolution. In SACLA, 19 5-m-long undulators (ID01-19) with 18 mm period are installed in the beamline [17] . The gap of each undulator can be independently controlled with the maximum K =2.15. 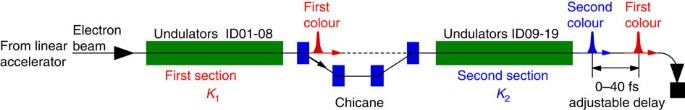Figure 1: Schematic layout of the SACLA undulator beamline. . Figure 1 is a schematic layout of the SACLA undulator beamline. After the eighth undulator (ID08), a magnetic chicane is installed to detour and retard the electron beam. The undulators are grouped into two sections before (ID01-08) and after (ID09-19) the chicane, and the undulator gaps of the two sections are simply set at different K values, K 1 and K 2 as in Figure 1 . Thus, two photon pulses emitted from the first section and the second section have different wavelengths, which are non-harmonic related. The temporal interval between the two pulses can be finely adjusted at resolution of attoseconds by changing the chicane parameters (see methods). The temporal pulse envelope of SASE is confirmed to be <10 fs (FWHM) by autocorrelation measurements [18] , [19] , which is consistent with the spectral spike widths observed by a single-shot spectrometer [20] . Figure 1: Schematic layout of the SACLA undulator beamline. . Full size image In the experiments, the electron beam was accelerated up to 7.8 GeV in a C-band linear accelerator and injected into the undulators. In the single-colour operation at 10 keV with K =2.1, the pulse energy of 250–300 μJ is routinely obtained with an intensity fluctuation of <10% as the relative s.d. [21] . Typical stabilities are around 3 × 10 −4 (s.d.) for the central wavelength and 0.1–0.2 μrad (s.d.) for the emission angle corresponding to 10% of the laser spot size. 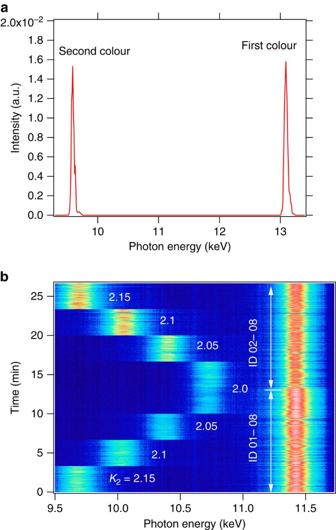Figure 2: Measured spectra of the two-colour XFEL. (a) Spectrum measured by scanning a monochromator withK1=1.7 andK2=2.15. (b) Consecutive single-shot spectra measured by an in-line spectrometer. The line at 11.4 keV is emitted from the first undulator section and the number of undulators is reduced from eight to seven at around 13 min on the ordinate.K2is varied stepwisely from 2.15 to 2.0 in the lower part and from 2.0 to 2.15 in the upper part of the figure. The accelerator was operated at 10 Hz and the sampling frequency of the in-line spectrometer was 1 Hz. Two-colour operation Figure 2a is the measured spectrum of the TCDP XFEL in which K 1 and K 2 were set at 1.7 (13.1 keV) and 2.15 (9.7 keV), respectively. In each undulator section, a slight gap taper was applied to compensate the beam energy loss due to resistive wakefields [17] . The spectrum was measured by scanning a monochromator and each data point was averaged over 100 shots. The pulse energy of 40 μJ was obtained for each photon energy. The relative wavelength separation of more than 30% was achieved as shown in Figure 2a . Figure 2: Measured spectra of the two-colour XFEL. ( a ) Spectrum measured by scanning a monochromator with K 1 =1.7 and K 2 =2.15. ( b ) Consecutive single-shot spectra measured by an in-line spectrometer. The line at 11.4 keV is emitted from the first undulator section and the number of undulators is reduced from eight to seven at around 13 min on the ordinate. K 2 is varied stepwisely from 2.15 to 2.0 in the lower part and from 2.0 to 2.15 in the upper part of the figure. The accelerator was operated at 10 Hz and the sampling frequency of the in-line spectrometer was 1 Hz. Full size image Figure 2b shows consecutive spectra during 30 min measured by a single-shot in-line spectrometer (see methods), which clearly present the stability and tunability of the TCDP operation. In Figure 2b , K 1 and K 2 were initially set at 1.9 (11.4 keV) and 2.15 (9.7 keV), respectively, for the first and second undulator sections. Then K 2 was first decreased from 2.15 to 2.0 by a 0.05 step from bottom to top in Figure 2b . Since the FEL gain becomes smaller for the smaller K 2 , the intensity of the second colour decreases as the photon energy increases. The number of the undulators of the first section was reduced from eight (ID01-08) to seven (ID 02-08) at the middle of Figure 2b , and then K 2 was increased to its initial value 2.15 by the same step. Whereas the intensity of the first colour (11.4 keV) drops with seven undulators, that of the second colour increases. In the TCDP operation, the electron beam energy spread resulting from the first-colour lasing affects the gain of the second colour [22] . 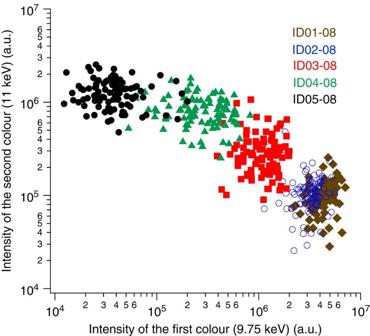Figure 3: Single-shot intensity correlation between the first and second colour pulses. The first colour is 9.75 keV (K1=2.14) and the second colour is 11 keV (K2=1.95). The symbol colours correspond to the different number of the first section undulators, eight undulators for brown diamonds, seven for blue open circles, six for red squares, five for green triangles and four for black solid circles. This relation is more clearly shown in Figure 3 , in which the shot-to-shot intensity correlation between the first and second colour pulses is plotted. K 1 and K 2 were set at 2.14 (9.75 keV) and 1.95 (11 keV), and the pulse energies were estimated from the integrated spectral area measured by the in-line spectrometer using a Gaussian fit (see methods). To vary the electron beam energy spread generated by the first-colour lasing, the number of the undulators of the first section was changed between eight (ID01-08) and four (ID05-08) by opening the undulator gaps. When all eight undulators were closed (brown diamonds in Fig. 3 ), the first-colour lasing was close to saturation. Under this condition, the pulse energy of the first colour (9.75 keV) was 140 μJ with a 23% fluctuation (s.d. ), whereas that of the second colour (11 keV) was a few μJ. The second-colour emission increases as decreasing the first-colour intensity by reducing the number of the undulators in the first section. The pulse energies of two colours can be balanced or relatively adjusted by changing the number of undulators. Figure 3: Single-shot intensity correlation between the first and second colour pulses. The first colour is 9.75 keV ( K 1 =2.14) and the second colour is 11 keV ( K 2 =1.95). The symbol colours correspond to the different number of the first section undulators, eight undulators for brown diamonds, seven for blue open circles, six for red squares, five for green triangles and four for black solid circles. Full size image Angular separation of two-colour pulses Since the amplification process of the second-colour pulse independently starts up from noise after the chicane, the electron density modulation at the first-colour wavelength or its smearing does not affect the lasing of the second-colour pulse. Thus, the second-colour pulse can be emitted on a completely different axis without losing the laser intensity. 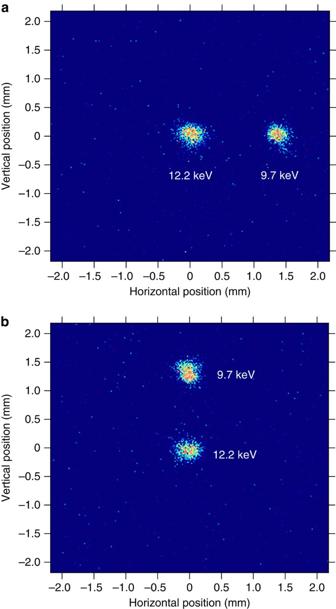Figure 4: Spatially separated two-colour pulses observed at 130 m downstream of the chicane. The first and second colours are 12.2 keV (K1=1.8) and 9.7 keV (K2=2.15), respectively. (a) The radiation axis of the second colour is horizontally deflected by 10 μrad. (b) The radiation axis of the second colour is vertically deflected by 10 μrad. In Figure 4 , K 1 and K 2 were set at 1.8 (12.2 keV) and 2.15 (9.7 keV), and the electron beam was deflected at the chicane by 10 μrad horizontally ( Fig. 4a ) and vertically ( Fig. 4b ). Two radiation profiles, each corresponding to the different photon energy, were observed on a diamond screen located 130 m downstream of the chicane. The pulse energies of 50 μJ and 31 μJ were obtained for 12.2 keV and 9.7 keV, respectively. To maintain a straight orbit of the electron beam, the undulator heights and the quadrupole magnet positions were accordingly aligned with respect to the deflected electron orbit downstream of the chicane. Note that the increase of the effective emittance due to a dispersion function [23] is negligibly small. Figure 4: Spatially separated two-colour pulses observed at 130 m downstream of the chicane. The first and second colours are 12.2 keV ( K 1 =1.8) and 9.7 keV ( K 2 =2.15), respectively. ( a ) The radiation axis of the second colour is horizontally deflected by 10 μrad. ( b ) The radiation axis of the second colour is vertically deflected by 10 μrad. Full size image The TCDP operation of XFEL realizes a jitter-free stable X-ray light source equipped with wide wavelength tunability of both colours and variable delay at attosecond resolution. In SACLA, the two colours are completely out of the SASE gain bandwidth to each other and the maximum wavelength separation of more than 30% has been achieved. The two-colour pulses can be separated not only spectrally but also spatially. The spatial separation enables the irradiation of the two-colour pulses from different angles to a sample. For example, simultaneous two-colour diffraction imaging from different angles becomes possible without losing photon intensity caused by a spectrometer. To improve longitudinal coherence, self-seeding techniques [24] , [25] can be applied to the TCDP XFEL by installing additional chicanes. Although further consideration is necessary, the TCDP operation combined with various methods of attosecond pulse generation [26] , [27] , [28] , [29] , [30] will make it feasible to study ultrafast phenomena, including coherent X-ray Raman scattering or hard X-ray atomic lasers, at an attosecond scale. Variable-gap undulator beamline The employment of fixed-gap undulators is a secure solution in terms of magnetic field errors, however it limits the tunability and flexibility of the XFEL operation, such as two-colour operation. Hence variable-gap in-vacuum undulators are adopted in SACLA. To avoid the magnetic field errors associated with the gap movement, synchrotron radiation from each undulator is utilized to check and correct the magnetic fields [17] . From its spectrum, K and height of the undulators are relatively aligned with the precision of 1.8 × 10 −4 (s.d.) and 10 μm (s.d. ), respectively. From its axis, the electron beam orbit of the undulator section is aligned along a straight line over 100 m. Together with feed-forward correction using a pair of steering coils, the overall straightness of the electron beam orbit is assured within ±10 μm at all operational undulator gaps, which is critically important to obtain overlap and interaction between the electron beam and radiation fields. In addition, the magnetic field quality of each undulator is routinely examined by the synchrotron radiation spectrum and an in situ field measurement system [31] . Time delay The length of the chicane installed in the SACLA undulator beamline is 5.1 m and the maximum delay is currently 40 fs limited by the capability of dipole magnets. Since the velocity of the electron bunch almost reaches the light velocity at relativistic energies, the time delay between the two photon pulses corresponds to the additional path length (Δ L ) of the electron beam at the chicane. The additional path length with respect to a straight trajectory is approximately given by Δ L ≈ θ 2 for a small deflection angle θ 1. L (=1.6 m) and L B (=0.3 m) are the drift distance between the first and second dipole magnets and the length of the magnet, respectively. Since the stabilities of the beam energy and the magnetic field, namely the deflection angle θ , are in the range of 10 −4 , the delay can be finely adjusted at precision of several tens of attoseconds. The transverse overlap of the two-colour pulses is assured by feed-forward orbit correction using a pair of steering magnets. The deviation of the electron beam orbit as a function of the delay is suppressed within ±5 μm downstream of the chicane. The maximum delay can be easily extended to a few hundreds of femtoseconds by replacing the dipole magnets. In-line spectrometer The in-line spectrometer monitors a part of Debye–Scherrer (111) diffraction rings from diamond powder using a multiport charge coupled device. Although the spectral resolution is limited to 100 eV at around 10 keV, which is larger than the SASE spectral width, it covers a single-shot spectral range of more than 2 keV. The pulse energies estimated from the integrated spectral area of the in-line spectrometer relatively agrees with a calibrated intensity monitor [32] within 2 × 10 −2 (s.d.) under the single-colour operation at 10 keV. How to cite this article: Hara, T. et al. Two-colour hard X-ray free-electron laser with wide tunability. Nat. Commun. 4:2919 doi: 10.1038/ncomms3919 (2013).